Solar steam generation by heat localization Currently, steam generation using solar energy is based on heating bulk liquid to high temperatures. This approach requires either costly high optical concentrations leading to heat loss by the hot bulk liquid and heated surfaces or vacuum. New solar receiver concepts such as porous volumetric receivers or nanofluids have been proposed to decrease these losses. Here we report development of an approach and corresponding material structure for solar steam generation while maintaining low optical concentration and keeping the bulk liquid at low temperature with no vacuum. We achieve solar thermal efficiency up to 85% at only 10 kW m −2 . This high performance results from four structure characteristics: absorbing in the solar spectrum, thermally insulating, hydrophilic and interconnected pores. The structure concentrates thermal energy and fluid flow where needed for phase change and minimizes dissipated energy. This new structure provides a novel approach to harvesting solar energy for a broad range of phase-change applications. Solar irradiation is a promising source of renewable energy, as the hourly incident solar flux on the surface of the earth is greater than annual global energy consumption [1] . Efficient harvesting of solar energy for steam generation is a key factor for a broad range of applications, from large-scale power generation, absorption chillers and desalination systems to compact applications such as water purification for drinking, sterilization and hygiene systems in remote areas where the only abundant energy source is the sun. Current methods of generating steam using solar energy rely on a surface or cavity to absorb the solar radiation, and transferring heat to the bulk liquid directly or via an intermediate carrier fluid, which require high optical concentration and suffer from high optical loss and surface heat loss [2] , [3] , [4] , or vacuum to reduce convective heat loss under moderate optical concentration. The steam thus generated is usually in thermal equilibrium with the bulk liquid. Nanofluids—fluids seeded with nanoparticles—as another alternative have been studied [5] , [6] , [7] as volumetric absorbers, potentially minimizing the surface energy loss by uniform temperature in the fluid [6] and enhanced thermal conductivity of nanofluid [8] , [9] . Local generation of steam in a cold bulk liquid can be achieved through high concentrations or illumination of nanofluids by electromagnetic waves (generally, lasers) with high power intensity [10] , [11] , [12] , [13] , [14] , [15] , [16] , [17] , [18] . Recently, Neumann et al . [7] , [19] succeed in generation of steam in bulk water with Au nanoparticles (NPs) with the power of 10 3 kW m −2 (optical concentration, C opt , of 1,000), consistent with the analysis of Phelan et al . [20] on several experiments concluding that Ag NPs with diameter of 20 nm had the lowest threshold light intensity for boiling at 2 × 10 3 kW m −2 . However, the solar thermal conversion efficiency of the approach was still only 24%. High optical concentrations limit the utilization of these approaches in stand-alone compact solar systems. Furthermore, high optical concentrations add complexity and cost to the solar thermal conversion system. We report the development of a new approach and corresponding material structure that localizes the solar energy where evaporation occurs and minimizes the heat losses leading to enhanced solar thermal efficiency at low optical concentration in open air while generating steam. As shown in Fig. 1a , under solar illumination, the developed structure forms a hot spot internally where evaporation occurs. The fluid wicks to the hot spot, evaporates and forms vapour which leaves the structure. This structure needs to have four main characteristics: high absorption in the solar spectrum, low thermal conductivity to suppress thermal conduction away from the hot internal region, hydrophilic surfaces to leverage capillary forces and promote fluid flow to the hot region, and interconnected pores for fluid flow to and from the structure. 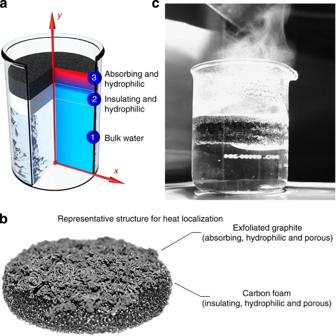Figure 1: Double-layer structure. (a) A representative structure for localization of heat; the cross section of structure and temperature distribution. (b) The DLS that consists of a carbon foam (10-mm thick) supporting an exfoliated graphite layer (~5-mm thick). Both layers are hydrophilic to promote the capillary rise of water to the surface. (c) A picture of enhanced steam generation by the DLS structure under the solar illumination of 10 kW m−2. Figure 1: Double-layer structure. ( a ) A representative structure for localization of heat; the cross section of structure and temperature distribution. ( b ) The DLS that consists of a carbon foam (10-mm thick) supporting an exfoliated graphite layer (~5-mm thick). Both layers are hydrophilic to promote the capillary rise of water to the surface. ( c ) A picture of enhanced steam generation by the DLS structure under the solar illumination of 10 kW m −2 . Full size image Material structure For the first demonstration of this approach, we developed a double-layer structure (DLS) consisting of a carbon foam layer supporting an exfoliated graphite layer ( Fig. 1b,c ). The bottom carbon foam is thermally insulating with smaller pore size for liquid supply and the top exfoliated graphite layer has larger pore size for vapour escape. Details of the DLS synthesis are given in the methods section. The optical transmission spectrum of the DLS is measured in the wavelength range of 200–1,500 nm ( Supplementary Fig. 1a ). The reflectivity of the exfoliated graphite is measured with a spectrophotometer equipped with an integrating sphere ( Supplementary Fig. 1b ) and it is <3% in the solar spectrum (250–2,250 nm). Thus, 97% of the irradiated solar power is absorbed within the top exfoliated graphite layer. The surface area of the exfoliated graphite layer is measured by N 2 adsorption to be approximately 320 m 2 g −1 , 32 times higher than graphite flakes for more efficient heat transfer to the fluid ( Supplementary Fig. 2 ). Receiver efficiency Solar absorption in the exfoliated graphite layer generates a hot region in the DLS. If fluid is constantly provided to this hot region, the evaporation rate reaches a steady-state condition. The experimental set-up for measurement of evaporation rate (and therefore efficiency) is shown in ( Supplementary Fig. 3 ). A test chamber is designed to assess performance of the DLS. This design is aimed to minimize two-dimensional and three-dimensional thermal losses. The thermal losses by the test chamber is simulated and discussed in ( Supplementary Fig. 4 ). The lab-scale size of the test chamber leads to a total of 6.5% parasitic losses, which can be avoided in large-scale applications ( Supplementary Note 4 ). Hence, higher receiver efficiency can be achieved in large systems. The evaporation rates of water with the DLS and the single exfoliated graphite layer (volumetric absorber) are measured by recording the weight change as a function of time and results are compared with pure water under solar illumination of 1 and 10 kW m −2 , Fig. 2a,b . After an initial transient period, the evaporation rate reaches a constant value. At each optical concentration, an experiment was run for a long illumination time (more than 5 h) and no change in evaporation rate is observed after the initial transient period. For pure water, the absorptance is small in the visible range. However, this small absorptance together with the larger absorptance in the infrared regime (not directly measured in this work) throughout the volume of the water causes an approximately 10 °C temperature rise in steady-state condition under a solar intensity of 1 kW m −2 . This temperature rise leads to enhanced evaporation (~6 times) compared with a dark environment ( Supplementary Fig. 5 ). The water evaporation rate in a dark environment is 74 kg m −2 h −1 . This ‘dark’ evaporation rate is subtracted from all the measured evaporation rates under the solar illumination to isolate the effect of solar irradiation on the evaporation rate. The DLS structure shows the highest evaporation rate and it is 2.1 and 2.4 times higher than pure water at 1 and 10 kW m −2 solar illumination, respectively. To show the effect of the bottom layer of the DLS, if only exfoliated graphite (volumetric absorber) is utilized, the evaporation rate drops by 17% due to heat losses by conduction to the underlying water. 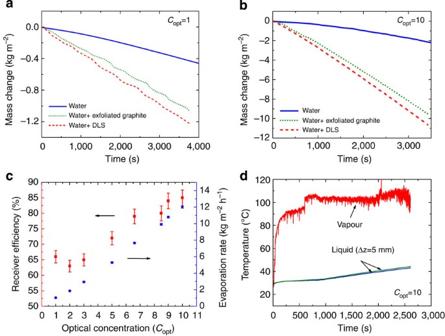Figure 2: Performance of the double-layer structure. The evaporation mass loss of water with different structures under (a) 1 kW m−2and (b) 10 kW m−2solar irradiation is compared with the case of pure water. All experiments are conducted in ambient temperature of 24 °C and the humidity of 31%. (c) The solar thermal efficiency of the evaporation process by the DLS under a range of optical concentrations (left-hand side axis) and the corresponding evaporation rate (right-hand side axis). (d) While the steam is generated, the underlying bulk liquid is at the ambient temperature. The thermal efficiency ( η th ) is considered to assess the performance of DLS and is defined as Figure 2: Performance of the double-layer structure. The evaporation mass loss of water with different structures under ( a ) 1 kW m −2 and ( b ) 10 kW m −2 solar irradiation is compared with the case of pure water. All experiments are conducted in ambient temperature of 24 °C and the humidity of 31%. ( c ) The solar thermal efficiency of the evaporation process by the DLS under a range of optical concentrations (left-hand side axis) and the corresponding evaporation rate (right-hand side axis). ( d ) While the steam is generated, the underlying bulk liquid is at the ambient temperature. Full size image where denotes the mass flux, h LV total enthalpy of liquid–vapour phase change (sensible heat+ phase-change enthalpy), C opt the optical concentration and q i the nominal direct solar irradiation 1 kW m −2 . The η th of the DLS is an increasing function of optical concentration and goes from 64% at 1 kW m −2 to 85% at 10 kW m −2 , Fig. 2c . We emphasize that optical concentration losses are not considered in this analysis. Note that this level of optical concentration can be achieved by simple non-imaging optics with monthly adjustment without a tracking system, which reduce the overall cost of the system. We calculate the conduction losses to the underlying water as described in ( Supplementary Figs 6 and 7 ). This loss at 10 kW m −2 is 5±0.5% of the total solar irradiation. The measured surface temperature of the exfoliated graphite is ~5 °C less than the generated vapour temperature. Considering emissivity of 0.97 ( Supplementary Fig. 1b ), under solar illumination of 10 kW m −2 , the radiation losses at the surface are 6%. At a solar irradiation of 1 kW m −2 , the fraction of losses is ~35% (reflection ~3%, conduction ~6%, surface radiation ~12%, test chamber parasitic losses ~14%). These losses are a decreasing function of solar irradiation, and the total loss drops to ~15% at 10 kw −2 . If the steam is generated with the DLS at higher concentrations, we expect that efficiencies of more than 90% is achievable. Here, we focused on low optical concentration to reduce the complexity and cost of solar-harvesting system. As a comparison, we have prepared a highly absorbing nanofluid with carbon-black NPs. The structures of NPs are shown in ( Supplementary Fig. 8 ). The sample preparation method is given in ( Supplementary Note 7 ). The nanofluid has absorption of >99% in the wavelength range of 250–2,250 nm. We have measured the receiver efficiency of this absorber with the same procedure used for the DLS ( Supplementary Fig. 9a ). The vapour generation rate by this type of receiver at solar irradiation of 10 kW m −2 is compared with the DLS in ( Supplementary Fig. 9b ). The nanofluid receiver leads to both lower vapour temperature (~80 °C) and lower efficiency compared with the DLS. The conversion efficiency of nanofluid receiver at solar irradiation of 10 kW m −2 is 75±3%, whereas this efficiency for the DLS is 85±3%. Furthermore, the fast dynamics of steam generation by the DLS is caused by heat localization at the liquid–vapour interface, making it a superior option in transient solar irradiation applications. The evaporation rate as a function of optical concentrations is also shown in Fig. 2c . Localized energy close to the surface of the structure accomponied by a limited flow rate of fluid leads to an enhanced temperature of the generated vapour phase. At 10 kW m −2 , while steam is generated, the underlying liquid is close to ambient temperature as shown in Fig. 2d . This non-equilibnrium process offers a localized phase-change, while the surrounding medium remains cold. This localization leads to a significant drop in thermal losses by the bulk fluid and consequently a boost in the thermal efficiency of solar thermal conversion. Note that our current system does not allow us to conduct experiments at higher pressures. Structure characterization Low thermal conductivities of the materials in the DSL structures are important for heat localization. We measured the thermal conductivity of each layer in this structure separately. The thermal conductivity of each layer is measured with an infrared (IR) microscope (See details in methods). In Fig. 3a–d , the thermal conductivity of each layer in air ( Fig. 3a,b ) and filled with water ( Fig. 3c,d ) are shown. The inset in each figure is a representative picture taken by an infrared (IR) microscope and indicates the temperature gradient across the sample. Since both structures are porous and have a large portion of air, their thermal conductivity is low in air. Once the exfoliated graphite (top layer) is filled with water, its thermal conductivity is larger than that of water and is not favourable for localizing heat, see Fig. 3c . However, the carbon foam shows a low thermal conductivity even when soaked in water. The carbon foam (bottom layer of the DLS) is critical for localizing thermal energy and the low thermal conductivity is due to the closed pores in this structure. These closed pores have three advantages: floating the structure, lowering the thermal conductivity and limiting the fluid flow to the surface. Low thermal conductivity and limited fluid flow lead to formation of a hot spot and generation of steam in the DLS at low optical concentrations. In contrast to closed pores, open pores provide paths for fluid to flow to the surface. 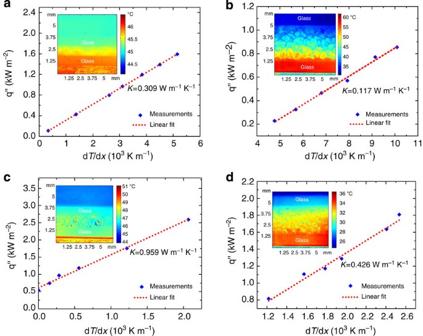Figure 3: Thermal conductivity of the double-layer structure. The thermal conductivity of each layer in the DLS is measured by an IR microscope (methods). (a) Exfoliated graphite in air, (b) carbon foam in air, (c) exfoliated graphite with water and (d) carbon foam filled with water. The inset in the figures are the representative picture taken by an IR microscope. Figure 3: Thermal conductivity of the double-layer structure. The thermal conductivity of each layer in the DLS is measured by an IR microscope (methods). ( a ) Exfoliated graphite in air, ( b ) carbon foam in air, ( c ) exfoliated graphite with water and ( d ) carbon foam filled with water. The inset in the figures are the representative picture taken by an IR microscope. Full size image The other important characteristic of the DLS is its hydrophilicity, which promotes fluid flow to the surface. The capillary force in the exfoliated graphite layer enhances the evaporation rate of the fluid through several mechanisms: formation of thin films on the surface of graphite sheets [21] , enhanced surface area for evaporation [22] and formation of three-phase contact lines at the edges of the capillaries [23] , [24] . The graphite structure has hydrophobic surfaces as evidenced by the contact angle ( Supplementary Fig. 10a ). However, after exfoliation in a microwave and oxidization of its surface, the graphite surface becomes hydrophilic ( Supplementary Fig. 10b ). The microstructure of graphite flakes before and after microwave exfoliation is presented in ( Supplementary Fig. 11 ). In practice, while the hydrophobic graphite flake appears dry on the water surface (see Fig. 4a ), the hydrophilic graphite flake results in formation of a thin layer of water on the top surface (see Fig. 4b ). The hydrophillic flakes leverage the capillary force to channel the fluid flow to the hot region. The microstructure of carbon foam is shown in ( Supplementary Fig. 12a ). The pores diameters are around 300–600 μm. Furthermore, the role of closed pores in floating the structure is highlighted in ( Supplementary Fig. 12b ) by comparing it with a carbon foam consisting of only open pores. In Fig. 4c , powdered carbon foam is dispersed on a water surface forming a dry surface indicating the hydrophobicity of this foam. To promote water flow, the carbon foam is treated by 4% molar nitric acid (see methods section), to make its surface hydrophilic, Fig. 4d . 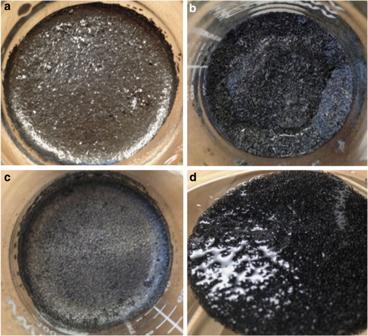Figure 4: Hydrophilicity of the double-layer structure. (a) The as-purchased graphite flakes possess hydrophobic surfaces and form a blanket over the water surface. (b) The synthesized graphite flakes are hydrophilic and form a thin layer of water on the surface. (c) The powdered carbon foam which is hydrophobic. (d) The processed carbon foam which is hydrophilic and promotes the capillary force and infiltration of water to the surface. Figure 4: Hydrophilicity of the double-layer structure. ( a ) The as-purchased graphite flakes possess hydrophobic surfaces and form a blanket over the water surface. ( b ) The synthesized graphite flakes are hydrophilic and form a thin layer of water on the surface. ( c ) The powdered carbon foam which is hydrophobic. ( d ) The processed carbon foam which is hydrophilic and promotes the capillary force and infiltration of water to the surface. Full size image Efficiency comparison To illustrate the insulating role of carbon foam, the underlying liquid temperature under the solar illumination of 1 kW m −2 is mesured for the DLS experiments and compared with just exfoliated graphite and pure water cases, as shown in Fig. 5a . Note that the thermocouples are shielded to eliminate the effect of direct solar illumination in the pure water experiments. As shown, the temperature of the water 15 mm below the water surface with the DLS structure is half of that in the other cases. In the absence of the bottom insulating foam, the temperature exceeds that of the pure water case due to a hot spot created in the exfoliated graphite layer. The generated vapour temperature with the DLS is measured under a range of optical concentrations and is plotted in Fig. 5b . With the DLS, steam >100 °C is generated at the solar illumination of 10 kW m −2 . A few degrees higher steam temperature than saturation temepearture at the ambient pressure is caused by the superheat required for hetrogeneous bubble nucleation. On the basis of the measured vapour temperature and evaporation mass flux, receiver efficiency of the DLS is determined for 1, 2 and 10 kW m −2 solar irradiation, Fig. 5c . At each solar concentration, this efficiency is compared with the receiver efficiency of water and single graphite layer on water. As shown, the DLS offers a high performance in solar thermal energy conversion compared with both cases. 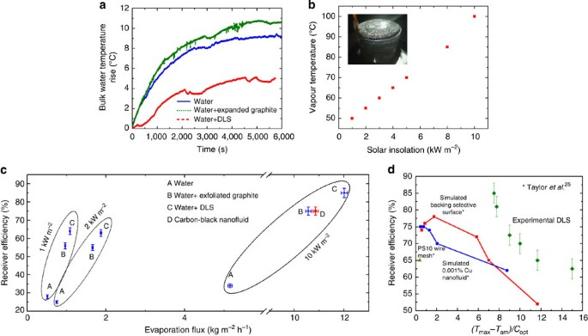Figure 5: Efficiency comparison. (a) The insulating behaviour of carbon foam is highlighted by measurement of underlying water temperature under 1 kW m−2and compared with other structures. For pure water, a radiation shield was installed on top of the thermocouple to eliminate the effect of direct radiation on the temperature reading. For the carbon structures, the transmittance of the structure is low enough that direct radiation does not contribute in temperature measurements. (b) The generated vapour temperature with the DLS under a range of optical concentrations. (c) The solar thermal conversion efficiency of the DLS is compared with water and single graphite layer under 1, 2, 10 kW m−2solar illumination. Furthermore, the receiver efficiency of a highly absorbing nanofluid is shown. The error bars in the efficiency values resulted from errors in the measurement of solar irradiation power and evaporation flux, and the error bars in the evaporation flux are resulted from error in the mass-change measurements. (d) The performance of DLS is compared with the current systems as a receiver in a solar tower collector25. All of these systems are non-vacuum, and no optical concentration losses are considered in these data. Figure 5: Efficiency comparison. ( a ) The insulating behaviour of carbon foam is highlighted by measurement of underlying water temperature under 1 kW m −2 and compared with other structures. For pure water, a radiation shield was installed on top of the thermocouple to eliminate the effect of direct radiation on the temperature reading. For the carbon structures, the transmittance of the structure is low enough that direct radiation does not contribute in temperature measurements. ( b ) The generated vapour temperature with the DLS under a range of optical concentrations. ( c ) The solar thermal conversion efficiency of the DLS is compared with water and single graphite layer under 1, 2, 10 kW m −2 solar illumination. Furthermore, the receiver efficiency of a highly absorbing nanofluid is shown. The error bars in the efficiency values resulted from errors in the measurement of solar irradiation power and evaporation flux, and the error bars in the evaporation flux are resulted from error in the mass-change measurements. ( d ) The performance of DLS is compared with the current systems as a receiver in a solar tower collector [25] . All of these systems are non-vacuum, and no optical concentration losses are considered in these data. Full size image Furthermore, the performance of the DLS is compared with some reported state-of-the-art systems [25] (selective absorbers, nanofluids and a type of volumetric absorber) and is presented in Fig. 5d . Note that all the systems are non-vacuum and no optical concentration losses are considered. These intrinsic efficiencies are plotted as a function of ( T max − T am )/ C opt where T max denotes maximum temperature of working fluid in the receiver and T am the ambient temperature ( Supplementary Note 7 ). As shown, DLS offers better performance than reported values of these systems and promises a new efficient approach for solar thermal harvesting. In addition, in the ( Supplementary Note 10 ) potential applications of the DLS are presented. In conclusion, we develop an approach and corresponding material structure, the DLS, which absorbs solar illumination, and confines the thermal energy (formation of hot spot) to near the structure surface while efficiently wicking the fluid to this hot spot. This structure yields a solar thermal conversion efficiency of 85% at 10 kW m −2 solar illumination, while generating steam in open air. Localization of heat is achieved by the broad-spectrum absorbing and thermally insulating properties of the DLS, while the fluid flow is channelled to the hot spot by the hydrophilic and porous nature of the DLS. We believe that by decreasing the flow rate in the carbon foam, replacing carbon foam with a more insulating material, and optimizing porosity and thickness of each layer (tuning capillary pressure in the sturucture) better performance such as higher steam temperature and/or at lower optical concentrations can be achieved. This work opens a new approach for solar-assisted steam generation for many potential applications. Synthesis of the DLS The acid-washed graphite flakes are obtained from Anthracite Industries. The acid-washed graphite flakes are mixed with the iron (II) acetate anhydrous, 97% (Strem Chemicals) with the ratio of 60–40 wt%. The mixture was heated in a microwave for 7 s to form an exfoliated fluffy structure [26] , [27] , [28] . The trapped gases between the graphite layers expand in the synthesis process and detach the flakes from each other. The volumetric exfoliation during this process is approximately 100 times. The dispersed iron species formed after the decomposition of iron (II) acetate provides a ferromagnetic structure. The ferromagnetism of the exfoliated graphite helps its collection after use. The acid-washed graphite flakes originally have a hydrophobic surface. However, in the exfoliation process, due to high temperature, the graphite surface is oxidized and turns into a hydrophilic surface. The Duocel carbon foam of type PPI 80 (80 pores per inch) is purchased from K. R. Reynolds. The carbon foam is washed in 4% molar nitric acid for 2 h under stirring to make its surface hydrophilic. Thermal conductivity measurements by IR microscope The thermal conductivity of each material is measured by sandwiching the material between two squared-shape glass slabs (reference materials) each 1-mm thick. The glass slabs are spaced from each other by double-stick tape and sealed in three sides for liquid measurements. The sandwich is placed between a heat source (Cu block heater) and a heat sink (thermoelectric cooler). The heat sink is maintained at a fixed temperature, while the current through the heat source is tuned to induce a range of temperature gradients across the sandwich. The whole structure is placed under an IR microscope. The emissivity map of the sandwich in an isothermal condition is first obtained followed by temperature distribution mapping. Since the thermal conductivity of reference materials is known, the measured temperature gradient in these materials is used to determine the heat flux. Given the heat flux, and measured temperature gradient in the material, the thermal conductivity of each material is calculated by the Fourier equation. The set-up is calibrated with water first and the measured thermal conductivity is within ±5% of the reported value. The linear correlation of heat flux and temperature gradient in Fig. 3 suggests a negligible contribution of convection side losses in the measurements. How to cite this article: Ghasemi, H. et al . Solar steam generation by heat localization. Nat. Commun. 5:4449 doi: 10.1038/ncomms5449 (2014).